Epigenomic profiling of primary gastric adenocarcinoma reveals super-enhancer heterogeneity Regulatory enhancer elements in solid tumours remain poorly characterized. Here we apply micro-scale chromatin profiling to survey the distal enhancer landscape of primary gastric adenocarcinoma (GC), a leading cause of global cancer mortality. Integrating 110 epigenomic profiles from primary GCs, normal gastric tissues and cell lines, we highlight 36,973 predicted enhancers and 3,759 predicted super-enhancers respectively. Cell-line-defined super-enhancers can be subclassified by their somatic alteration status into somatic gain, loss and unaltered categories, each displaying distinct epigenetic, transcriptional and pathway enrichments. Somatic gain super-enhancers are associated with complex chromatin interaction profiles, expression patterns correlated with patient outcome and dense co-occupancy of the transcription factors CDX2 and HNF4α. Somatic super-enhancers are also enriched in genetic risk SNPs associated with cancer predisposition. Our results reveal a genome-wide reprogramming of the GC enhancer and super-enhancer landscape during tumorigenesis, contributing to dysregulated local and regional cancer gene expression. Aberrant gene expression patterns are a universal hallmark of human malignancy driving clinically important traits such as proliferation, invasion and metastasis [1] . Cancer transcriptomes can be reprogrammed by genomic alterations (somatic mutations, copy number alterations and structural variations) affecting signalling molecules and transcription factors (TFs) [2] . Besides protein-coding genes, cis -regulatory elements in noncoding genomic regions can also influence transcriptional programs by facilitating or restricting TF accessibility [3] . Distinct regulatory element classes are defined by different epigenomic marks, involving DNA methylation, histone methylation/acetylation and other combinations [4] . For example, promoters are marked by histone H3 lysine 4 tri-methylation (H3K4me3), enhancers by H3K4me1, active regulatory elements by H3K27ac and repressive features by H3K27me3 [5] , [6] . A growing number of studies are now highlighting the significance of histone modifications in the development and maintenance of disease states [4] , [6] , [7] . It has also been proposed that because epigenetic modifications are more stable than RNA transcripts, histone modification profiling may offer a better measure of transcriptional status than RNA sequencing [8] . Enhancers are regulatory elements localized distal to promoters and transcription start sites (TSSs). Occupying 10–15% of the human genome [9] , enhancers play important roles in cell identity and tissue-specific expression by regulating one or more genes at large distances (>1 Mb) [10] . Recent studies have demonstrated that enhancers can be subdivided into different classes, with one such class comprising enhancer clusters occurring in close proximity, referred to as ‘super-enhancers’ [11] , [12] . Compared to typical enhancers, super-enhancers are larger in size, exhibit higher TF binding densities and are strongly associated with key cell identity regulators, similar to locus control regions [13] , DNA methylation valleys [14] , transcription initiation platforms [15] and stretch enhancers [16] . Super-enhancers are also enriched in disease-associated genetic variants [11] , are acquired by cancer cells at key oncogenes [11] , and importantly are more sensitive to therapeutic perturbation [12] . The emerging importance of super-enhancers in human disease, coupled with their exquisite tissue-specificity, raises a need for comprehensive super-enhancer catalogues of different cell types and disease conditions. In cancer, such super-enhancer catalogues are indeed emerging, for both haematological and solid malignancies [11] , [17] . However, most of these studies to date have relied on in vitro cultured cancer cell lines, which have two limitations. First, in vitro cell lines are known to experience substantial epigenomic alterations after repeated passaging [18] . Second, for many cancer cell lines, matched normal counterparts are frequently not available, complicating the ability to identify true tumor-specific somatic alterations. Gastric cancer (GC) is the fifth most common cancer worldwide and the third leading cause of global cancer mortality [19] . Most GCs are adenocarcinomas, and molecular studies have revealed key genetic alterations associated with gastric malignancy, including mutations in chromatin modifier genes such as ARID1A , and amplifications in HER2 , FGFR2 and MET [20] . In contrast to genetic alterations, our knowledge of the GC epigenome remains poorly understood, with current knowledge largely confined to patterns of aberrant DNA methylation [21] . To address the role of histone modifications in GC, we recently reported a proof-of-concept study employing micro-scale chromatin profiling (Nano-ChIPseq) to survey histone modifications in primary GCs [4] . In this study, we extended this effort to characterize the GC super-enhancer landscape. By integrating predicted super-enhancer data from both cell lines and primary tumours, we provide evidence that like enhancers, predicted super-enhancers are heterogeneous and can be further subclassified into biologically distinct subgroups with impact on tumour-specific gene expression, cancer hallmarks and disease genetic variation. We also found that in GCs, predicted super-enhancers exhibiting somatic gain are associated with CDX2 and HNF4α occupancy. Taken collectively, our results reveal a pervasive reprogramming of the gastric super-enhancer landscape during tumourigenesis, underpinning wide-spread alterations in cancer gene expression. Distal predicted enhancer landscapes of GC cell lines Using Nano-ChIPseq, we generated 110 chromatin profiles from 19 primary GCs, 19 matched normal gastric tissues and 11 GC cell lines covering multiple histone H3 modifications (H3K27ac, H3K4me3, H3K4me1) (average ∼ 3.3 × 10 7 reads per profile). 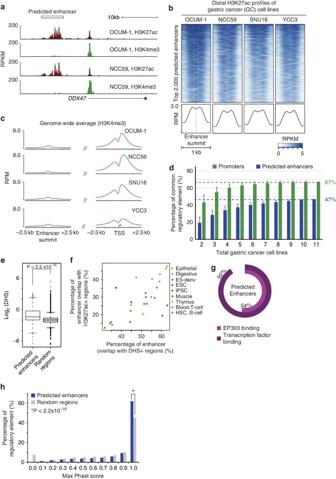Figure 1: Distal Predicted Enhancer landscapes of GC cell lines. (a) Histone profiles of OCUM-1 and NCC59 GC cells show enrichment of H3K27ac and H3K4me3 around theDDX47TSS. A predicted enhancer element exhibiting H3K27ac enrichment and >2.5 kb away from theDDX47TSS was identified. (b) Snapshot of distal H3K27ac profiles in 4 of the 11 GC cell lines, visualizing the activity of the top 2,000 predicted enhancers and the genome-wide average H3K27ac signal around the predicted enhancers. (c) Genome-wide average H3K4me3 signals around predicted enhancers and active TSSs in GC cell lines. (d) Recurrence rates of regulatory elements. Data presented are the mean percentage +/− standard deviation of common regulatory elements (enhancer—blue; promoter—green) found in two or more gastric cancer cell lines, as a function of number of cell lines. (e) Chromatin accessibility of predicted enhancers versus randomly selected regions. DNase I hypersensitivity (DHS) data from normal gastric tissues28was used as a surrogate. The distribution of DHS signals was tested using a one-side Welch’st-test for statistical significance. (f) Percentage of overlap between predicted enhancers, chromatin accessible regions (denoted as DHS+,xaxis) and active regulatory elements (denoted as H3K27ac+,yaxis) from 50 epigenomic profiles originating from nine different tissue/cell categories. (g) Percentage of predicted enhancers overlapping with EP300 and transcription factor binding sites. (h) Distribution of maximum Phast scores (a measure of DNA sequence conservation) in predicted enhancers and randomly selected regions. 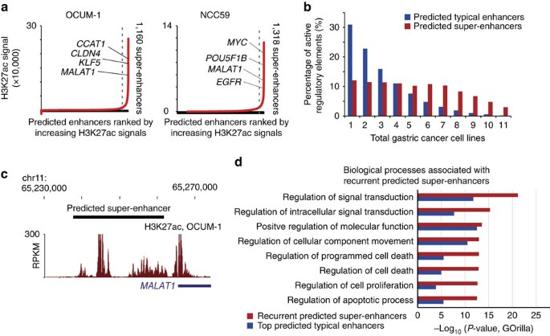Figure 2: GC cell-line-derived predicted super-enhancers. (a) Distribution of H3K27ac ChIP-seq signals reveal locations of predicted super-enhancers showing unevenly high H3K27ac signals. Known cancer-associated genes proximal to predicted super-enhancers are indicated. Two cell lines are shown. (b) Percentage of distal regulatory elements (predicted typical enhancers—blue, predicted super-enhancers—red) showing H3K27ac enrichment above randomly selected regions (>99%) across increasing numbers of GC cell lines. (c) H3K27ac ChIP-seq signals at theMALAT1locus shows stretches of predicted enhancers, corresponding to a predicted super-enhancer (in filled box) with high H3K27ac signals. (d) Examples of top significantly associated biological processes associated with recurrent distal regulatory elements (predicted super-enhancers and top predicted typical enhancers). Negative log-transformed rawP-values from GOrilla were used. Clinical information and molecular classification of the primary GCs is presented in Supplementary Table 1 , sequencing statistics in Supplementary Data 1 and clinico-pathological details for the GC lines in Supplementary Table 2 . Our series included 10 gland forming adenocarcinomas (53%, intestinal type), 6 samples with highly infiltrating isolated cells (32%, diffuse type) and 3 GC samples (15%) of mixed histology. More than 60% of the tumours ( n =12) were Stage 3 or above (AJCC 7th edition). We performed extensive quality control analysis of the Nano-ChIPseq data, including variations in mapping quality filters, analysis of biological replicates and promoter ChIP-enrichment, and assessment by the quality control software CHANCE (CHip-seq ANalytics and Confidence Estimation [22] ). Increasing mapping threshold stringencies (from MAPQ ≥10 to 20) did not appreciably alter mapping statistics: >90% of the total mapped reads were retained, and 85% of ChIP-enriched peaks and 98% of predicted enhancers were rediscovered respectively ( Supplementary Fig. 1 ). Histone peak concordance between biological replicates of KATO-III cells generated by Nano-ChIPseq, and also against independent KATO-III H3K27ac data generated by conventional ChIP-seq [23] , confirmed high reproducibility (overlaps of ∼ 85 and ∼ 90%) ( Supplementary Fig. 2 ). Comparisons of input and input-corrected H3K27ac and H3K4me3 signals at 1000 promoters associated with highly expressed protein-coding genes revealed successful enrichment in 48 out of 50 (96%) H3K27ac and 42 out of 42 (100%) H3K4me3 libraries respectively. CHANCE analysis of ChIP enrichment, particularly for H3K4me1 (which is depleted at promoters), revealed that the large majority (85%) of samples exhibited successful enrichment (Methods). These results demonstrate the good technical quality of the Nano-ChIPseq cohort. Besides Nano-ChIPseq, the samples were also processed for DNA methylation analysis (Infinium HumanMethylation 450 K BeadChip arrays), copy number analysis (Affymetrix SNP arrays) and Illumina RNA-sequencing. We chose to use GC cell lines as a discovery cohort to discover cancer-associated distal enhancers in GC, as cell lines are purely epithelial in nature, have the highest data quality, and because previous studies have shown that stromal contamination in primary tissues can influence genomic results [24] . We also focused on recurrent epigenetic alterations present in multiple GC samples, which reduces the introduction of ‘private’ epigenetic alterations associated with individualized cell line features. First, we mapped genome-wide cis -regulatory elements based on H3K27ac signals, previously shown to mark active promoters and enhancers [4] . To enrich for enhancer elements, we focused on H3K27ac signals located distant from known annotated TSSs (TSSs; >2.5 kb) in accordance with previous studies [25] ( Fig. 1a ). We then further refined the enhancer predictions using aggregated H3K4me1 and H3K4me3 data, excluding from analysis predicted enhancers exhibiting high H3K4me3/H3K4me1 log ratios (>2.4) [26] . Using this approach, we identified 3,017 to 14,338 putative distal enhancers in the GC lines ( Fig. 1b ), with an average genomic footprint of 25 Mb/line. Figure 1: Distal Predicted Enhancer landscapes of GC cell lines. ( a ) Histone profiles of OCUM-1 and NCC59 GC cells show enrichment of H3K27ac and H3K4me3 around the DDX47 TSS. A predicted enhancer element exhibiting H3K27ac enrichment and >2.5 kb away from the DDX47 TSS was identified. ( b ) Snapshot of distal H3K27ac profiles in 4 of the 11 GC cell lines, visualizing the activity of the top 2,000 predicted enhancers and the genome-wide average H3K27ac signal around the predicted enhancers. ( c ) Genome-wide average H3K4me3 signals around predicted enhancers and active TSSs in GC cell lines. ( d ) Recurrence rates of regulatory elements. Data presented are the mean percentage +/− standard deviation of common regulatory elements (enhancer—blue; promoter—green) found in two or more gastric cancer cell lines, as a function of number of cell lines. ( e ) Chromatin accessibility of predicted enhancers versus randomly selected regions. DNase I hypersensitivity (DHS) data from normal gastric tissues [28] was used as a surrogate. The distribution of DHS signals was tested using a one-side Welch’s t -test for statistical significance. ( f ) Percentage of overlap between predicted enhancers, chromatin accessible regions (denoted as DHS+, x axis) and active regulatory elements (denoted as H3K27ac+, y axis) from 50 epigenomic profiles originating from nine different tissue/cell categories. ( g ) Percentage of predicted enhancers overlapping with EP300 and transcription factor binding sites. ( h ) Distribution of maximum Phast scores (a measure of DNA sequence conservation) in predicted enhancers and randomly selected regions. Full size image In total, we detected 36,973 predicted distal enhancer regions, spanning ∼ 140 Mb or approximately 5% of the human genome. The predicted enhancers exhibited a bimodal H3K27ac signal distribution [11] ( Fig. 1b ), were depleted of H3K4me3 and were enriched in H3K4me1 signals, similar to enhancer modification profiles reported in previous studies [6] ( Fig. 1c and Supplementary Fig. 3 ). Visual comparison of selected H3K27ac-enriched regions revealed that some regions are active in multiple lines (‘recurrent’) while other regions are active in only one line (‘private’). These observations are similar to previous results in both lymphoblastoid [27] and colon carcinoma cell lines [7] . Approximately 47% of the predicted enhancers were recurrent, exhibiting activity in at least two GC cell lines ( Fig. 1d ). The percentage of recurrent enhancers was significantly lower compared to promoters (67 versus 47%, P <2.2 × 10 −16 , one-sided proportion test), indicating that enhancer activity is highly variable across GC cell lines. We validated the predicted enhancers by integrating publicly available epigenomic datasets. Using DNase I hypersensitivity (DHS) data of normal gastric tissues from the Epigenome Roadmap, we found that DHS signal distributions (log-transformed RPKM) at predicted enhancers were significantly greater than randomly selected regions ( P <2.2 × 10 −16 , one-sided Welch’s t -test; Fig. 1e , Methods), indicating that predicted enhancers are associated with open chromatin. When compared against DHS and H3K27ac data of nine different tissue and cellular categories [28] , predicted enhancers exhibited the highest overlap with DHS-positive and H3K27ac-positive regions from digestive and epithelial tissues (fetal intestine, gastric and small intestine), and were distinct from non-epithelial tissue types such as blood and T-cells ( Fig. 1f ). Supporting their regulatory potential, 54% of the predicted enhancers ( n =20,127) were associated with EP300 binding sites ( Fig. 1g ; P <0.001, empirical test), and 92% with TF binding sites. At the DNA sequence level, 63% of the predicted enhancer sequences were evolutionarily conserved ( Fig. 1h ; P <0.0001, empirical test). Super-enhancers are enriched in cancer signatures ‘Super-enhancers’ or ‘stretch-enhancers’ refer to a sub-population of enhancers displaying extended physical proximity (+/− 12.5 kb), and have been proposed to be critical for cell identity and maintenance of healthy or disease state [11] , [12] . Using the ROSE algorithm [12] , we identified 133 to 1318 predicted super-enhancers per GC line, collectively encompassing 3,759 non-redundant-predicted super-enhancers ( Fig. 2a ). We thus estimate that about 10% of GC cell-line-predicted enhancers are associated with predicted super-enhancer activity, consistent with the 4–19% estimated by other studies [11] . Compared to predicted typical enhancers, predicted super-enhancers exhibited a significantly greater tendency to be recurrent ( Fig. 2b ; one-sided proportion test, P <2 × 10 −16 ), with 3,345 predicted super-enhancers being active in at least two GC cell lines. We observed predicted super-enhancers associated with known protein-coding GC oncogenes (for example, MYC and KLF5; Supplementary Fig. 4a ) and also at non-protein-coding gene regions such as at the MALAT1 locus ( Fig. 2c ), which encodes a long-noncoding RNA (lncRNA) recently shown to promote GC proliferation [29] . Figure 2: GC cell-line-derived predicted super-enhancers. ( a ) Distribution of H3K27ac ChIP-seq signals reveal locations of predicted super-enhancers showing unevenly high H3K27ac signals. Known cancer-associated genes proximal to predicted super-enhancers are indicated. Two cell lines are shown. ( b ) Percentage of distal regulatory elements (predicted typical enhancers—blue, predicted super-enhancers—red) showing H3K27ac enrichment above randomly selected regions (>99%) across increasing numbers of GC cell lines. ( c ) H3K27ac ChIP-seq signals at the MALAT1 locus shows stretches of predicted enhancers, corresponding to a predicted super-enhancer (in filled box) with high H3K27ac signals. ( d ) Examples of top significantly associated biological processes associated with recurrent distal regulatory elements (predicted super-enhancers and top predicted typical enhancers). Negative log-transformed raw P -values from GOrilla were used. Full size image We assigned predicted super-enhancers to target genes based on regions exhibiting the nearest active TSS (defined as H3K27ac enrichment at promoters, within 500 bp of an annotated TSS). This strategy has been previously used in other studies [11] . Consistent with other reports [26] , only 53% of our predicted super-enhancer/gene interactions involved the closest proximal gene (see Methods, mean distance 76 kb). We validated the predicted super-enhancer/gene assignments using three orthogonal interaction data sets: (i) pre-determined interactions predicted by PreSTIGE [30] , (ii) GREAT [31] , and (iii) published RNAPII ChIA-PET data (encodeproject.org, GSE72816). Of 2,677 predicted interactions with protein-coding genes, 88% were supported by at least one of these three data sets ( Supplementary Fig. 5 ). This number is likely a lower limit as the biological samples for the latter validation data in (i)-(iii) did not involve gastric tissues (see subsequent sections). To understand biological themes associated with the predicted super-enhancers, we applied GOrilla pathway analysis [32] and found that biological processes plausibly related to cancer development, such as regulation of signal transduction, programmed cell death and cell proliferation were strongly associated with predicted super-enhancer linked genes ( P -values 6.7 × 10 −22 to 2.3 × 10 −13 , hypergeometric test by GOrilla) ( Fig. 2d ). Many of these processes (eg, regulation of programmed cell death, cell proliferation) remained significantly associated when the recurrent predicted super-enhancers were analysed by GREAT, indicating that that these enrichments are not due to biases toward genes flanked by large intergenic regions ( Supplementary Fig. 6 ). Similar analyses employing genes linked to the top predicted typical enhancers yielded a lesser degree of enrichment ( Fig. 2d ). Predicted super-enhancer associated genes were also enriched for oncogenes ( P =1.7 × 10 −8 , one-sided Fisher’s exact test). When correlated to gene expression, genes associated with recurrent predicted super-enhancers and typical enhancers were both significantly correlated with RNA expression ( Supplementary Fig. 4b ). Super-enhancer heterogeneity in primary tumours To determine which cell-line-predicted super-enhancers are also associated with somatic alterations in vivo , we compared H3K27ac enrichment levels for these regions across 19 primary GCs and matched normal gastric tissues. While previous studies have suggested the presence of distinct molecular subtypes of GC [33] , [34] , [35] , due to limited sample sizes we elected in the current study to focus on predicted enhancer differences conserved in multiple GC tissues relative to matched normal tissues (see Discussion). Prior to analysis, we confirmed that the primary gastric normal samples were indeed reflective of gastric epithelia, by correlating against published profiles ( Supplementary Discussion ). Of 3,759 cell-line-predicted super-enhancers, two-thirds exhibited differential enrichment between tumours and matched normal samples ( Fig. 3a , Supplementary Data 2 , referred to as somatically altered thereafter). Close to half of the predicted super-enhancers ( n =1748; 47%) exhibited somatic gain in two or more primary GCs (> 2-fold enrichment in tumour, minimum 0.5 RPKM difference), and principal component analysis (PCA) using these gained predicted super-enhancers confirmed separations between GC and matched normal tissues ( Fig. 3b ). Supporting the consistency of these results, the vast majority of these recurrent somatic gain predicted super-enhancers (85%, >1.5-fold change threshold) were rediscovered when using only those normal/tumour (N/T) primary pairs passing all quality control criteria (14 pairs, see earlier). Unexpectedly, despite their activity in cancer cell lines, a substantial proportion of predicted super-enhancers (18%) were associated with somatic loss rather than gain in primary GCs ( Fig. 3a ). It is possible that these latter regions may represent regions epigenetically silenced in primary tumours but reactivated in cell lines during in vitro culture ( Supplementary Fig. 7a ). In all, 11% of the predicted super-enhancers ( n =416) exhibited unaltered H3K27ac levels between GCs and normal tissues ( Fig. 3a , Supplementary Fig. 7b ), consistent with these regions not being cancer-associated but related to ‘housekeeping’ or general tissue functions. Finally, 21% ( n =808) of cell-line-predicted super-enhancers did not exhibit sufficient H3K27ac enrichment (RPKM<0.5) in primary samples for analysis ( Supplementary Fig. 7c ). Interestingly, this class was also associated with low recurrence in GC lines ( Fig. 3a —histogram in black). Taken collectively, these results demonstrate that predicted super-enhancers derived from cell lines can be further subclassified using histone modification data from primary tumours and matched normal controls into at least three categories—somatic gain, somatic loss and unaltered. A list of the top 100 somatic predicted super-enhancers is presented in Supplementary Data 2 . 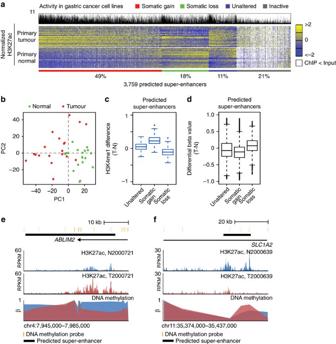Figure 3: Somatic predicted super-enhancers in primary GCs and matched normal samples. (a) Activity of cell-line-derived predicted super-enhancers in 19 primary tumour and matched normal samples. H3K27ac predicted super-enhancer signals in units of column-transformed RPKM values (z-score) were visualized. The frequency of active predicted super-enhancers in GC linesin vitrois presented as the top histogram (black, above the heatmap). Predicted super-enhancers were categorized into somatic gain, somatic loss, unaltered and inactive. In each category, the predicted super-enhancers were ordered (left to right) by their decreasing mean difference between the tumour and the normal samples. (b) Principal component analysis using recurrent somatic gain predicted super-enhancer signals establish a separation between tumour and normal samples. (c) Differences in H3K4me1 (T-N) signals (RPKM) using H3K4me1 profiles from five tumour and matched normal samples in three predicted super-enhancer categories: somatic gain, somatic loss and unaltered. *P<2.2 × 10−16, one-sided Welcht-test. (d) Differentialβvalues in predicted super-enhancers indicate the state of methylation: hypermethylation (>0) or hypomethylation (<0) between tumours and matched normal samples. (e) DNA hypomethylation in a somatic gain predicted super-enhancer at theABLIM2locus. (f) DNA hypermethylation in a somatic loss predicted super-enhancer at theSLC1A2locus. Figure 3: Somatic predicted super-enhancers in primary GCs and matched normal samples. ( a ) Activity of cell-line-derived predicted super-enhancers in 19 primary tumour and matched normal samples. H3K27ac predicted super-enhancer signals in units of column-transformed RPKM values ( z -score) were visualized. The frequency of active predicted super-enhancers in GC lines in vitro is presented as the top histogram (black, above the heatmap). Predicted super-enhancers were categorized into somatic gain, somatic loss, unaltered and inactive. In each category, the predicted super-enhancers were ordered (left to right) by their decreasing mean difference between the tumour and the normal samples. ( b ) Principal component analysis using recurrent somatic gain predicted super-enhancer signals establish a separation between tumour and normal samples. ( c ) Differences in H3K4me1 (T-N) signals (RPKM) using H3K4me1 profiles from five tumour and matched normal samples in three predicted super-enhancer categories: somatic gain, somatic loss and unaltered. * P <2.2 × 10 −16 , one-sided Welch t -test. ( d ) Differential β values in predicted super-enhancers indicate the state of methylation: hypermethylation (>0) or hypomethylation (<0) between tumours and matched normal samples. ( e ) DNA hypomethylation in a somatic gain predicted super-enhancer at the ABLIM2 locus. ( f ) DNA hypermethylation in a somatic loss predicted super-enhancer at the SLC1A2 locus. Full size image Supporting their biological distinctiveness, predicted super-enhancers belonging to the three categories also exhibited other epigenetic differences in vivo . For example, predicted super-enhancer alterations in H3K27ac were similarly correlated with H3K4me1 enhancer mark alterations ( Fig. 3c ), and at the DNA methylation level somatic gain predicted super-enhancers exhibited significantly lower DNA methylation levels, while somatic loss super-enhancers exhibited increased DNA methylation ( P =3.8 × 10 −229 , one-sided Welch’s t -test). Unaltered predicted super-enhancers occupied an intermediate range ( Fig. 3d ). As a visual example, we observed decreased DNA methylation (indicated by a lower beta value) in GC T2000721 compared to its matched normal (N2000721), mapping to a somatic gain predicted super-enhancer at the ABLIM2 locus ( Fig. 3e ). In contrast, somatic loss of H3K27ac signals at a SLC1A2 predicted super-enhancer in T2000639 showed increased DNA methylation compared to N2000639 ( Fig. 3f ). These results further support the biological and molecular heterogeneity of predicted super-enhancers in gastric tissues. Super-enhancers exhibit complex chromatin interactions Integration with copy number data revealed that the majority of somatic predicted super-enhancers are localized to copy number neutral regions ( Supplementary Fig. 8a-c , Supplementary Discussion ). To examine associations between predicted super-enhancers and gene expression, we interrogated RNA-seq information from the same primary samples, using the same predicted super-enhancer/gene assignments as the previous pathway analyses ( Fig. 2 ). Somatic gain predicted super-enhancers were associated with elevated gene expression relative to matched normal samples, while somatic loss predicted super-enhancers were associated with decreased expression ( P <2.2 × 10 −16 , one-sided Welch t -test; Fig. 4a ). 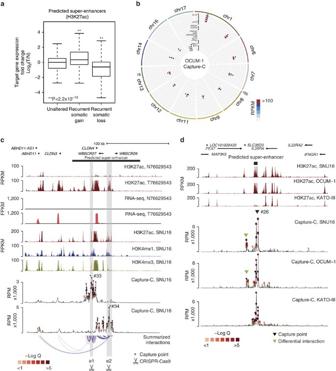Figure 4: Associations between somatic predicted super-enhancers with gene expression and chromatin interactions. (a) Correlation between log-transformed fold changes in gene expression between different classes of predicted super-enhancers (unaltered, somatic gain, somatic loss) and predicted target gene expression. (b) Interaction heat map from 20 capture points covering 12 somatic gain predicted super-enhancers. Each ring represents a profile from a single capture point, denoted by a black arrowhead. Locations of the predicted super-enhancers are indicated by the gene loci in each ring. Genome-wide interaction signals were computed across the genome in 100 kb bins. Signals at regions within 2 million bases flanking the capture points were visualized. (c) Example of a somatic gain predicted super-enhancer at theCLDN4locus and interactions with neighbouring genes. Somatic gain activity is associated with upregulation ofCLDN4and neighbouring genes (CLDN3andABHD11) in primary GCs. Interactions were detected in SNU16 cells using two capture points, #33 and #34 by Capture-C. Summarized interactions (Q<0.05, r3Cseq) are presented as the last track. Two constituent predicted enhancers, e1 and e2, were deleted independently in SNU16 cells using CRISPR/Cas9 genome editing. (d) Correlation between predicted super-enhancer activity and long-range interactions. Long-range interactions (green triangle) to theSLC35D3promoter were detected with a predicted super-enhancer active in SNU16 and OCUM-1 cells. Such interactions were not observed in KATO-III cells where the predicted super-enhancer was also not detected. Figure 4: Associations between somatic predicted super-enhancers with gene expression and chromatin interactions. ( a ) Correlation between log-transformed fold changes in gene expression between different classes of predicted super-enhancers (unaltered, somatic gain, somatic loss) and predicted target gene expression. ( b ) Interaction heat map from 20 capture points covering 12 somatic gain predicted super-enhancers. Each ring represents a profile from a single capture point, denoted by a black arrowhead. Locations of the predicted super-enhancers are indicated by the gene loci in each ring. Genome-wide interaction signals were computed across the genome in 100 kb bins. Signals at regions within 2 million bases flanking the capture points were visualized. ( c ) Example of a somatic gain predicted super-enhancer at the CLDN4 locus and interactions with neighbouring genes. Somatic gain activity is associated with upregulation of CLDN4 and neighbouring genes ( CLDN3 and ABHD11 ) in primary GCs. Interactions were detected in SNU16 cells using two capture points, #33 and #34 by Capture-C. Summarized interactions ( Q <0.05, r3Cseq) are presented as the last track. Two constituent predicted enhancers, e1 and e2, were deleted independently in SNU16 cells using CRISPR/Cas9 genome editing. ( d ) Correlation between predicted super-enhancer activity and long-range interactions. Long-range interactions (green triangle) to the SLC35D3 promoter were detected with a predicted super-enhancer active in SNU16 and OCUM-1 cells. Such interactions were not observed in KATO-III cells where the predicted super-enhancer was also not detected. Full size image Previous research has also shown that enhancers are often involved in long-range chromatin interactions that may influence the expression of multiple genes [10] , [26] . To identify long-range interactions associated with somatic predicted super-enhancers in GC, we applied Capture-C technology [36] to survey interactions for 36 predicted super-enhancers, selected from regions exhibiting both recurrent somatic gains in primary tumour samples and also demonstrating activity in GC lines. Analysing three GC cell lines (OCUM-1, SNU16, KATO-III), we probed multiple genomic locations ( n =92, referred to as ‘capture points’) across the 36 predicted super-enhancers, identifying 88 capture points with significant interactions ( Q <0.05, r3Cseq package [37] ). Fig. 4b depicts 12 representative predicted super-enhancers covering 20 capture points. On average, each predicted super-enhancer exhibited 20–26 and 5–7 interactions with other genomic locations and promoters respectively. The average distance between capture points and detected interactions was approximately 17.0 kb (standard deviation: 30.5 kb). We also identified longer-range interactions, including a predicted super-enhancer interaction with the TM4SF4 promoter at a distance of ∼ 100 kb in OCUM-1 cells ( Supplementary Fig. 9 ). Notably, for regions with informative interaction data, the availability of experimental Capture-C information also allowed us to further validate 93% ( n =62) of our original predicted super-enhancer/gene interactions. Integration of expression data from the cell lines revealed that ∼ 70% of the interacting promoters are associated with detectable gene expression (FPKM>0). As a representative example, Fig. 4c depicts the long-range interaction landscape of the CLDN4 genomic region in SNU16 cells (see Supplementary Fig. 10 for other examples). This region was selected as CLDN4 expression has been previously associated with GC progression and prognosis [38] , and recurrent gain of the CLDN4 predicted super-enhancer was observed in multiple primary GCs ( Supplementary Fig. 8d ). Specifically, we sought to investigate interactions involving two predicted sub-super-enhancer regions exhibiting high H3K27ac signals and also CDX2 and HNF4α co-binding (see later). Besides interactions with the CLDN4 promoter, interactions were also detected with other distal promoters (up to ∼ 100 kb) such as WBSCR27 , CLDN3, ABHD11 and ABHD11-AS1 . ABHD11-AS1 is a long non-coding RNA was previously shown to be highly expressed in gastric cancer [39] . To validate the Capture-C data, we also performed circularized chromosome conformation capture assays (4C) [40] on four selected predicted super-enhancers in two GC lines (OCUM-1, SNU16) ( Supplementary Fig. 11 ). We observed a concordance between Capture-C and 4C data of 75%, similar to concordance rates between 4C experimental replicates [37] ( Supplementary Fig. 12 ). Due to the significantly greater depth of 4C sequencing, we also identified additional interactions, such as a long-range interaction between a predicted super-enhancer and the KLF5 promoter at a distance of ∼ 350 kb ( Supplementary Fig. 11b ). Previous reports have suggested that certain long-range interactions are associated with super-enhancer activity, while other interactions are more invariant and reflective of cell lineage [10] , [41] . In agreement with these findings, of 22 (out of 36) predicted super-enhancers displaying differential activity between the GC lines, four predicted super-enhancers exhibited a good correlation between predicted super-enhancer activity and the presence of long-range interactions ( Fig. 4d and Supplementary Fig. 13 ). For the remaining 18 predicted super-enhancers, long-range interactions were observed independent of predicted super-enhancer activity. To investigate a causal role between the predicted super-enhancers and gene expression, we used CRISPR/Cas9 genome editing to delete two enhancer regions (e1 and e2; see Fig. 4c ) within the CLDN4 predicted super-enhancer region. After confirming CRISPR deletion efficiencies in OCUM-1 and SNU16 cells ( Supplementary Fig. 14a–c ), we compared predicted target gene expression levels between enhancer-deleted and wild-type cells by RT-qPCR. In both cell lines, e1 CRISPR-deletion caused downregulation of multiple CLDN4 locus genes, including ABHD11 , CLDN3 and CLDN4 ( CLDN4 in SNU16 cells, Supplementary Fig. 14d ). In a similar fashion, we also observed ABHD11 , CLDN3 and CLDN4 downregulation after e2 deletion in OCUM-1 cells (e2-deleted SNU16 cells were not viable, hence precluding gene expression analysis; Supplementary Fig. 14e ). To extend these results, we then CRISPR deleted two other predicted enhancer elements (e3 and e4) from the ELF3 predicted super-enhancer in OCUM-1 cells ( Supplementary Figs 11a and 14c ), as ELF3 has been reported as a cancer gene in several malignancies [42] . Both e3 and e4 deletion resulted in downregulation of multiple ELF3 locus genes including ARL8A, ELF3, RNPEP and TIMM17A ( Supplementary Fig. 14f ). Taken collectively, these results support a causal relationship between predicted super-enhancer activity and tumour gene expression. Somatic super-enhancers and clinical outcome To further explore the biological and clinical relevance of predicted super-enhancer heterogeneity, we performed cancer hallmark analysis categorized by somatic modification status (gained, lost, unaltered). Of ten cancer hallmarks [11] , somatic gain predicted super-enhancers were significantly enriched in genes related to invasion ( P =8.6 × 10 −11 , one-sided Fisher’s exact test), angiogenesis ( P =2.4 × 10 −4 , one-sided Fisher’s exact test) and cell death resistance ( P =7.8 × 10 −3 , one-sided Fisher’s exact test), exceeding somatic loss and predicted unaltered super-enhancers by an order of magnitude ( Fig. 5a ). These results suggest that somatic gain predicted super-enhancers may be involved in traits associated with aggressive GC. When compared against predicted super-enhancer profiles of 86 cell and tissue samples, >60% of somatic gain predicted super-enhancers in GC exhibited high tissue-specificity. We also observed significant overlaps ( P <0.001, empirical test) with predicted super-enhancers previously described in other cancer types, such as colorectal, breast, cervical and pancreatic cancer ( Supplementary Fig. 15 ), suggesting that certain GC-associated predicted super-enhancers may also be active in other cancer types. 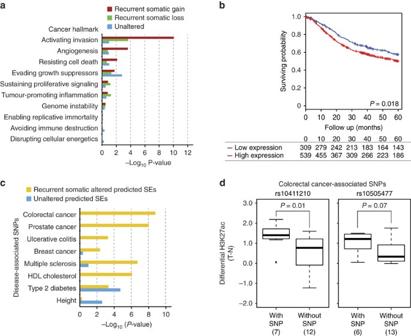Figure 5: Somatic predicted super-enhancers inform patient survival and disease risk. (a) Cancer hallmark analysis using predicted super-enhancers showing recurrent somatic gain, recurrent somatic loss and unaltered H3K27ac signals. Negative log-transformedP-values from the one-sided Fisher’s exact test were used. (b) Survival analysis comparing patient groups with samples exhibiting low (blue) and high (red) expression from genes associated with top recurrent somatic gain predicted super-enhancers. The signature is prognostic in the compilation of 848 GC patients (P=1.8 × 10−2, log-rank test), with worse prognosis observed for patients with tumours having high signature expression (hazard ratio, 95% confidence interval: 1.30 (1.05–1.61); Cox regressionP-value after correcting for stage, age, patient locality and Lauren’s histological subtypes=4.4 × 10−2). Survival data are indicated for every 10 months. (c) Enrichment of disease-associated SNPs in predicted super-enhancers. Enrichments were tested on two classes of predicted super-enhancers: recurrent somatic altered and unaltered predicted super-enhancers using chi-square test. Only diseases/traits with at least 10 SNPs found in all predicted super-enhancers were analysed. (d) Differential H3K27ac signals in predicted super-enhancers with and without colorectal cancer associated SNPs. The total number of patients with or without the SNPs is indicated in brackets. The difference between the two groups was tested using one-sided Welcht-test. Figure 5: Somatic predicted super-enhancers inform patient survival and disease risk. ( a ) Cancer hallmark analysis using predicted super-enhancers showing recurrent somatic gain, recurrent somatic loss and unaltered H3K27ac signals. Negative log-transformed P -values from the one-sided Fisher’s exact test were used. ( b ) Survival analysis comparing patient groups with samples exhibiting low (blue) and high (red) expression from genes associated with top recurrent somatic gain predicted super-enhancers. The signature is prognostic in the compilation of 848 GC patients ( P =1.8 × 10 −2 , log-rank test), with worse prognosis observed for patients with tumours having high signature expression (hazard ratio, 95% confidence interval: 1.30 (1.05–1.61); Cox regression P -value after correcting for stage, age, patient locality and Lauren’s histological subtypes=4.4 × 10 −2 ). Survival data are indicated for every 10 months. ( c ) Enrichment of disease-associated SNPs in predicted super-enhancers. Enrichments were tested on two classes of predicted super-enhancers: recurrent somatic altered and unaltered predicted super-enhancers using chi-square test. Only diseases/traits with at least 10 SNPs found in all predicted super-enhancers were analysed. ( d ) Differential H3K27ac signals in predicted super-enhancers with and without colorectal cancer associated SNPs. The total number of patients with or without the SNPs is indicated in brackets. The difference between the two groups was tested using one-sided Welch t -test. Full size image We next asked if gene expression patterns associated with the somatic gain predicted super-enhancers might be associated with GC patient survival. We selected genes associated with the top 50 predicted super-enhancers, from regions exhibiting both recurrent somatic gains in multiple GC patients, and also exhibiting the highest correlations with target gene expression. Supporting the validity of this approach, several genes selected in this manner were observed to have been previously shown to be overexpressed in GC, such as CDH17 [43] and CCAT1 [44] . The gene list also included potentially novel GC associated genes, such as SMURF1 and LINC00299 ( Supplementary Table 3 ). We performed survival analysis across three non-Asian GC and four Asian GC cohorts comprising of 848 GC patients. Patients with GCs exhibiting high expression of predicted super-enhancer associated genes showed poor overall survival compared with GC samples where these genes are relatively lowly expressed ( Fig. 5b , P =1.8 × 10 –2 , log rank test). Supporting the robustness of this association, the relationship with patient survival remained significant even after varying the number of predicted super-enhancers ( n =30, P =0.02, log rank test; n =60, P =0.03, log rank test). In a multivariate analysis, the association with survival also remained statistically significant even after adjusting for other risk factors, such as age, stage, patient locality and histological subtype ( P =0.044, Wald test). These data indicate that genes driven by somatic gain predicted super-enhancers in GC may be clinically important. To address the relationship between the different predicted super-enhancer categories and disease risk, we considered previous genome-wide association studies (GWAS) studies showing that disease-associated single-nucleotide polymorphisms (SNPs) are enriched at regulatory elements [11] , [45] . We mapped catalogues of disease-associated SNPs reported from 1,470 GWAS against those predicted super-enhancers exhibiting recurrent somatic alterations (gained or lost) or unaltered predicted super-enhancers. Somatic predicted super-enhancers were enriched for disease-risk SNPs associated with various cancers (prostate, colorectal, breast; enrichment ratio=3.0–7.2; P <4.4 × 10 −3 , chi-square test) and gastrointestinal diseases such as ulcerative colitis (enrichment ratio=3.3; P =5.2 × 10 −4 , chi-square test) ( Fig. 5c ). In contrast, unaltered predicted super-enhancers did not exhibit similar enrichments. Unexpectedly, we also observed enrichment of multiple sclerosis SNPs in somatic altered predicted super-enhancers (enrichment ratio=4.3; P =1.8 × 10 −7 , chi-square test), suggestive of interconnections between cancer and autoimmune response [46] . To explore if predicted super-enhancer disease SNPs might be associated with local changes in chromatin modification, we then focused on SNPs associated with colorectal cancer reported in at least two studies and also exhibiting heterozygosity in at least 1/3 of the GC patients (see Discussion). Two SNPs fulfilled these criteria (rs10411210 and rs10505477). Samples with the rs10411210 SNP exhibited significantly higher H3K27ac signals in tumours versus matched normals ( Fig. 5d ; P =0.01, one-sided Welch’s t -test), and a similar trend was also observed in samples with the rs10505477 SNP ( P =0.07, one-sided Welch’s t -test). Such associations suggest a relationship between disease-associated risk SNPs and cancer-associated histone modification. Super-enhancers exhibit dense TF occupancy Finally, we explored trans -acting factors associated with somatic gain predicted super-enhancers. Concordant with previous studies [47] , GC predicted super-enhancers exhibited significantly enriched ENCODE TF binding profiles compared to other genomic regions, supporting the former as TF ‘hot-spots’ ( P <2.2 × 10 −16 , one-sided proportion test). Interrogating the ReMap database [48] , we then identified specific TFs associated with the different predicted super-enhancer categories. Both somatic gain and unaltered predicted super-enhancers exhibited enrichments in CEBPB, MYC and FOXA1 binding. However, among the top ten enriched TFs, CDX2 exhibited elevated enrichment in somatic gain predicted super-enhancers (rank #2), with an approximately 30% increased binding density compared to unaltered predicted super-enhancers (rank #8) ( Fig. 6a,b ). 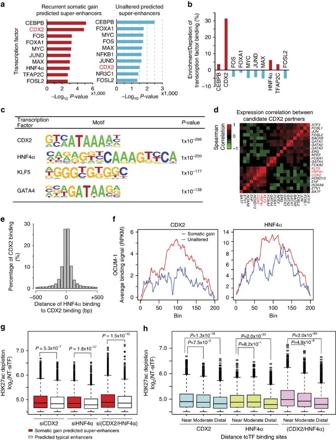Figure 6: Somatic gain predicted super-enhancers in GC are associated with CDX2 and HNF4α occupancy. (a) Top 10 transcription factor binding enrichments at recurrent somatic gain predicted super-enhancers and unaltered predicted super-enhancers using the ReMap database. (b) Enrichment or depletion of ReMap transcription factors at recurrent somatic gain predicted super-enhancers compared to unaltered predicted super-enhancers. (c) Detection of candidate CDX2 binding partners using CDX2 binding sites andde novoHOMER motif identification. (d) Pairwise expression correlations of CDX2 and top 20 CDX2 candidate binding partners using RNA-seq from 19 primary tumour and matched normal samples. (e) Percentage of CDX2 binding sites co-occurring with HNF4α binding sites within a 500 bp window in OCUM-1 cells. (f) Differential CDX2 (left) and HNF4α (right) average binding signal analysis between recurrent somatic gain predicted super-enhancers and unaltered predicted super-enhancers. The predicted super-enhancers were also active in OCUM-1. (g) Distribution of H3K27ac depletion magnitude in between somatic gain predicted super-enhancers and predicted typical enhancers in OCUM-1 cells, for single and double TF silencing. Statistical significance was evaluated using the one-sided Wilcoxon rank sum test. (h) Association between H3K27ac sub-regional depletion in somatic gain predicted super-enhancers relative to CDX2, HNF4α or CDX2/HNF4α co-binding sites. Distances were uniformly distributed into three categories: near, moderate and distal to the binding sites. Statistical significance was evaluated using one-sided Wilcoxon rank sum test. Figure 6: Somatic gain predicted super-enhancers in GC are associated with CDX2 and HNF4α occupancy. ( a ) Top 10 transcription factor binding enrichments at recurrent somatic gain predicted super-enhancers and unaltered predicted super-enhancers using the ReMap database. ( b ) Enrichment or depletion of ReMap transcription factors at recurrent somatic gain predicted super-enhancers compared to unaltered predicted super-enhancers. ( c ) Detection of candidate CDX2 binding partners using CDX2 binding sites and de novo HOMER motif identification. ( d ) Pairwise expression correlations of CDX2 and top 20 CDX2 candidate binding partners using RNA-seq from 19 primary tumour and matched normal samples. ( e ) Percentage of CDX2 binding sites co-occurring with HNF4α binding sites within a 500 bp window in OCUM-1 cells. ( f ) Differential CDX2 (left) and HNF4α (right) average binding signal analysis between recurrent somatic gain predicted super-enhancers and unaltered predicted super-enhancers. The predicted super-enhancers were also active in OCUM-1. ( g ) Distribution of H3K27ac depletion magnitude in between somatic gain predicted super-enhancers and predicted typical enhancers in OCUM-1 cells, for single and double TF silencing. Statistical significance was evaluated using the one-sided Wilcoxon rank sum test. ( h ) Association between H3K27ac sub-regional depletion in somatic gain predicted super-enhancers relative to CDX2, HNF4α or CDX2/HNF4α co-binding sites. Distances were uniformly distributed into three categories: near, moderate and distal to the binding sites. Statistical significance was evaluated using one-sided Wilcoxon rank sum test. Full size image As TFs often act in a cooperative manner, we then identified potential CDX2 partners by using HOMER [49] , a de novo motif discovery algorithm. HOMER analysis identified HNF4α, KLF5 and GATA4 binding motifs associated with CDX2 binding ( Fig. 6c ). We also analysed CDX2 co-binding motifs using PScanChIP [50] with JASPAR 2016. Using PScanChIP, we predicted 367 proteins as potential CDX2 partners, once again including HNF4α, KLF5 and GATA4 ( Supplementary Data 3 ). Gene co-expression analysis revealed that HNF4 α (Spearman correlation, r =0.80) and KLF5 ( r =0.58) are the most strongly correlated candidates with CDX2 expression, suggesting that HNF4α and KLF5 may be likely CDX2 partners ( Fig. 6d ). Notably, CDX2 has been previously identified in GC as a driver of intestinal metaplasia [51] , and KLF5 and GATA4/6 have been previously reported as oncogenic TFs in GC that cooperate to upregulate HNF4 α [52] . To experimentally confirm genomic co-occupancy of CDX2 with HNF4α (the highest correlated factor), we performed CDX2 and HNF4α ChIP-seq on OCUM-1 gastric cells, and integrated the TF binding locations with predicted super-enhancer locations. In OCUM-1 cells, CDX2 and HNF4α binding summits ( q <0.01, MACS2) exhibited high co-occurrence (500 bp window), with 76% of CDX2 binding co-occurring with HNF4α (known as CDX2/HNF4α sites) ( Fig. 6e ). Comparing the top 50% of high CDX2 -expressing GCs against the lowest 50%, we found that in the former samples, recurrent somatic gain predicted super-enhancers were indeed associated with higher CDX2 binding densities (123 bindings per million base pair, Mbp versus 92 Mbp; see Methods). CDX2/HNF4α sites were preferentially localized to somatic gain predicted super-enhancers relative to unaltered predicted super-enhancers ( P =2.4 × 10 −4 , chi-square test), and both CDX2 and HNF4α binding signals were increased at somatic gain predicted super-enhancers relative to unaltered predicted super-enhancers ( Fig. 6f ). Similar CDX2 and HNF4α ChIP-seq results were also obtained in SNU16 cells ( Supplementary Fig. 16a ). This result indicates that somatic gain predicted super-enhancers in GC are associated with CDX2 and HNF4α occupancy. To test if CDX2 and HNF4α might play a role in GC super-enhancer maintenance, we performed silencing of each TF, either singly or both factors simultaneously, followed by genome-wide H3K27ac profiling. Depletion of either factor, either individually or in combination, did not induce global changes in H3K27ac in OCUM-1 cells ( Supplementary Fig. 16b ). However, CDX2 and HNF4 α-silencing led to specific H3K27ac alterations in 9.7 Mb and 4.3 Mb of the genome respectively, and double-TF knockdown induced significantly greater H3K27ac depletion ( P =3.4 × 10 −29 and 1.2 × 10 −88 compared to CDX2 and HNF4 α-alone, one-sided Wilcoxon rank sum test) ( Supplementary Fig. 16c ). For both single-TF and double-TF silencing, H3K27ac depletion occurred more prominently at somatic gain predicted super-enhancers compared to predicted typical enhancers, suggesting a heightened sensitivity of super-enhancer activity to TF depletion ( Fig. 6g , Supplementary Fig. 16d , Supplementary Data 4 ; P =5.3 × 10 −7 ; P =1.8 × 10 −17 ; P =1.5 × 10 −10 for CDX2 , HNF4 α and CDX2/HNF4 α respectively, one-sided Wilcoxon rank sum test). Supporting the specificity of these effects, H3K27ac depletion at predicted super-enhancers was more pronounced at regions centred at CDX2 or HNF4α binding sites, particularly at sites co-occupied by both factors ( Fig. 6h ). Similar results were also obtained in SNU16 cells ( Supplementary Fig. 16e ). Next, to assess relationships between predicted super-enhancers and gene expression, we focused on predicted super-enhancers exhibiting H3K27ac depletion after TF silencing. We observed that >60% of predicted super-enhancer target genes also exhibited reduced expression after TF silencing (si CDX2 , P =4 × 10 −4 , empirical test; si HNF4 α, P <1 × 10 −4 , empirical test; si( CDX2/HNF4 α), P <1 × 10 −4 , empirical test; Supplementary Fig. 16f ). This proportion significantly exceeded that expected by chance, as assessed by permutation analysis (Methods). Taken collectively, these results support a functional requirement for CDX2 and HNF4α in GC super-enhancer maintenance. GC is a clinically heterogeneous disease, and besides surgery and chemotherapy, only traztuzumab (anti-HER2) and ramucirumab (anti-VEGFR2) are approved clinically with other molecularly targeted agents proving unsuccessful to date [20] . Epigenomic deregulation has emerged as an important pathway in gastric tumorigenesis, with chromatin modifier genes (eg, ARID1A ) being frequently mutated in GC [53] , [54] and epigenetic alterations associated with gastric pre-malignancy [55] . To date however, the vast majority of GC epigenomic studies have focused on promoter DNA methylation in the context of tumour suppressor gene silencing (for example, CDH1 , RUNX3 ). In contrast, very little is currently known about distal regulatory elements (that is, enhancers) in GC. Here, we analysed >35k predicted enhancer elements identified through micro-scale histone modification profiling of primary gastric tumours, matched non-malignant tissues and GC cell lines. Small-scale ChIP protocols are known to be technically challenging and may sometimes result in significant between-sample variability. Reassuringly, we have previously demonstrated that Nano-ChIP signals between tumours and normal samples exhibit a good concordance with orthogonal ChIP-qPCR results [4] and in the present study we also performed extensive quality control analyses, including variations in mapping stringency, biological replicate analysis, promoter ChIP enrichment and CHANCE analysis, to confirm that the vast majority (85–100%) of our Nano-ChIPseq libraries are of acceptable quality. Our focus on recurrent epigenomic alterations present in multiple samples further ensured that our biological conclusions are likely to be robust, as shown by the observation that 84% of the recurrent somatic gain predicted super-enhancers were still rediscovered when analysis was confined to only those ‘high-quality’ tumour/normal pairs passing both promoter-based and CHANCE quality analysis. Nevertheless, we also note there is still scope for improving the data quality of such experiments, such as using spike-in approaches to better ascertain inter-experimental variations or to exclude extreme experiments [56] . Our study was motivated by recent studies in other cancer types demonstrating a fundamental role for distal enhancers and super-enhancers in cell identity and disease [7] , [11] , [16] , [25] , [45] . Indeed, in our study and others [11] , recurrent predicted super-enhancers largely manifested at known oncogenes and genes participating in oncogenic processes ( Fig. 2d ). We also observed high levels of enhancer variation between individual samples, exceeding proximal promoter elements ( Fig. 1d ). When compared against other tissues and tumour-types, almost 60% of GC predicted super-enhancers were tissue-specific ( Supplementary Fig. 15 ). It is worth noting that in the current study we studied GCs as a general category against matched non-malignant gastric tissues for maximal sensitivity; however, recent studies have highlighted distinct histopathological and molecular GC subtypes [33] , [34] , [35] . Indeed, a preliminary analysis comparing recurrent somatic gain predicted super-enhancers between 10 intestinal and 6 diffuse GCs identified 471 and 224 predicted super-enhancers specific to intestinal- and diffuse-type GCs respectively, and 516 common predicted super-enhancers. These results also suggest that there may exist distinct enhancer alterations in different histological subtypes of GC. Such findings reflect the exquisite tissue-specific nature of enhancer elements, and the consequent need for generating comprehensive enhancer catalogues in expanded patient cohorts and in many different tumour types. The majority of samples analysed in our study were primary tissues derived directly from patients, rather than in vitro cultured cell lines. By comparing predicted enhancer activities (H3K27ac) between tumours and matched normals, we were able to further sub-classify cell line predicted super-enhancers according to their somatic alteration status (somatic gain, somatic loss and unaltered). Supporting their biological distinctiveness, the subcategorized predicted super-enhancers also displayed specific differences in other orthogonal features, including epigenomic patterns (H3K4me1, DNA methylation), gene transcription and cancer hallmarks. Notably, in our data only a small fraction of somatic gain predicted super-enhancers localized to regions of copy number amplification. Our results thus complement recent studies implicating focal amplification as a mechanism for super-enhancer activity in cancer [57] . The ability to subclassify predicted super-enhancers according to bona-fide somatic gain or loss is likely to improve downstream attempts to pinpoint oncogenic mechanisms responsible for establishing super-enhancers in cancer. Such approaches are also possibly extendable to other disease states [45] . A priori consideration of predicted super-enhancer heterogeneity may also prove useful when analysing germline variants associated with disease risk. While previous findings have reported that disease-associated SNPs are generally over-represented in regulatory elements [7] , [9] , [11] , we found that somatic altered, but not unaltered predicted super-enhancers, were specifically enriched in SNPs associated with cancer and inflammatory gastrointestinal disease (a known risk factor for gastrointestinal cancer). SNPs in these regions may alter disease risk and cancer development through several non-exclusive mechanisms, including modification of TF binding motifs [58] , regulation of long-range chromatin interactions [26] or alteration of H3K27ac levels. Indeed, in our study, we observed that two SNPs associated with colorectal cancer (CRC) risk (rs10505477 and rs10411210) [59] were also associated with local changes in chromatin modification in primary GCs. There are several reasons why it may be plausible to integrate CRC risk data with GC. First, at least one of these CRC risk SNPs (rs10505477) has been reported to also influence GC clinical outcome in both treatment response and patient survival [60] . Second, the key TFs associated with the GC predicted super-enhancers ( CDX2 , HNF4 α) are also known to regulate colonic development [61] , [62] . Third, the role of intestinal metaplasia (IM) as a pre-malignant risk factor for GC is well-established, and in IM the gastric epithelial cells adopt a cellular architecture and appearance similar to colonic epithelium [20] . The observation that these genetic variants, while present in germline DNA, may influence chromatin structure and gene expression in the tumour has also been observed in CRC [63] . These results further highlight the importance of studying aberrant epigenetic states to refine our understanding of germline processes underlying disease predisposition. Our results suggest certain general principles regarding how individual super-enhancers in GC might interact with the cis- and trans- acting transcriptional machinery. Using two distinct long-range chromatin interaction assays (Capture-C and 4C), we observed several examples of somatic gain predicted super-enhancers engaging both proximal and distal genes exhibiting elevated tumour expression. It has been proposed that genes linked to somatic gain predicted super-enhancers are likely to occupy similar topological associating domains, established through cohesin-mediated enhancer-promoter loops [64] . The ability of somatic gain predicted super-enhancers to influence both proximal and distal gene expression implicates predicted super-enhancers as pivotal regulators of aberrant gene expression in gastric tumours, which can contribute to disease progression and chemoresponse [35] ( Fig. 5b ). At the trans - level, our data revealed that somatic gain predicted super-enhancers in GC are associated with CDX2 and HNF4α occupancy. Previous studies have shown that aberrant CDX2 expression in the stomach is associated with intestinal metaplasia of the mucosal epithelial cells, an important early event in gastric tumour formation and that CDX2 has the potential to function as a GC oncogene [65] . HNF4α has also been recently implicated in GC, as a target of both the lineage-specific oncogenes KLF5 and GATA factors [52] , and the AMPK signalling pathway [20] . Our results in primary human tumours are supported by recent findings in the mouse small intestine, where CDX2 has been found to regulate HNF4α occupancy to control intestinal gene expression [66] . Echoing these studies, we also found that CDX2/HNF4α depletion effected chromatin alterations at local regions concentrated at CDX2 and/or HNF4α binding sites. A potential limitation in our study is that the modest albeit significant differences in H3K27ac observed after TF silencing may be due to use of transient knockdown compared to stable gene silencing. While it is thus possible that CDX2 and HNF4α may influence GC super-enhancer activity in a more wide-spread manner, these results nevertheless support a specific role for CDX2 and HNF4α in GC predicted super-enhancer maintenance. In conclusion, our study demonstrates a role for heterogeneity in predicted super-enhancers and the utility of intersecting chromatin profiles from primary tissues and cell lines to dissect regulatory biology. This first-generation roadmap of GC distal enhancers now renders possible future integrative studies involving transcriptional features associated with GC predicted enhancers (eRNAs), and identifying somatic regulatory mutations perturbing predicted super-enhancer activity [67] . We also note that in this study, we have focused on heterogeneity between patients; however, intra-tumour heterogeneity is also emerging as an important mechanism of GC treatment resistance [68] . Future studies should be focused on investigating the role of epigenetic deregulation in GC intra-tumour heterogeneity. Taken collectively, these studies will likely deepen our knowledge of GC enhancer biology and regulatory circuits underlying this deadly malignancy. Primary tissue samples and cell lines Primary patient samples were obtained from the SingHealth tissue repository with approvals from the SingHealth Centralised Institutional Review Board and signed patient informed consent. ‘Normal’ (that is, non-malignant) samples used in this study refers to samples harvested from the stomach, from sites distant from the tumour and exhibiting no visible evidence of tumour or intestinal metaplasia/dysplasia upon surgical assessment. Tumour samples were confirmed by cryosectioning to contain >40% tumour cells. FU97, MKN7, OCUM-1 and RERF-GC-1B cell lines were obtained from the Japan Health Science Research Resource Bank. KATO-III and SNU16 cells were obtained from the American Type Culture Collection. NCC-59 was obtained from the Korean Cell Line Bank. YCC3, YCC7, YCC21, YCC22 were gifts from Yonsei Cancer Centre, South Korea. Cell line identities were confirmed by STR DNA profiling performed at the Centre for Translational Research and Diagnostics (Cancer Science Institute of Singapore, Singapore). STR profiles were assessed according to the standard ANSI/ATCC ASN-0002-2011 nomenclature, and the profiles of our cell lines showed >80% similarity to the reference databases. MKN7 cells—one commonly misidentified line by ICLAC ( http://iclac.org/databases/cross-contaminations/ ) was confirmed by showing a perfect match (100%) with the MKN7 reference profile in the Japanese Collection of Research Bioresources Cell Bank. MycoAlert Mycoplasma Detection Kits (Lonza) and MycoSensor qPCR Assay Kits (Agilent Technologies) were used to detect mycoplasma contamination. All cell lines were negative for mycoplasma contamination. For this study, we selected OCUM-1 and SNU16 cells as our main cell line models for two reasons. First, OCUM-1 and SNU16 cells were originally isolated from patients with poorly differentiated GC, and the majority of primary GCs in our study are poorly differentiated (63%). Second, OCUM-1 and SNU16 have been previously used as GC models in many other published studies [69] , [70] , and are thus regarded as accepted GC models in the field. Thus, OCUM-1 and SNU16 were used as consistent cell line models for several experiments, including Capture-C, 4C, enhancer CRISPR, TF binding and TF knockdown. Nano ChIPseq Nano-ChIPseq was performed as described [4] with slight modifications. For primary tissues, fresh-frozen cancer and normal tissues were dissected using a razor blade in liquid nitrogen to obtain ∼ 5 mg sized piece for each ChIP. Tissue pieces were fixed in 1% formaldehyde/PBS buffer for 10 min at room temperature. Fixation was stopped by addition of glycine to a final concentration of 125 mM. Tissue pieces were washed three times with tris buffered saline with EDTA (TBSE) buffer. For cell lines, 1 million fresh harvested cells were fixed in 1% formaldehyde/medium buffer for 10 min at room temperature. Fixation was stopped by addition of glycine to a final concentration of 125 mM. Fixed cells were washed three times with TBSE buffer, and centrifuged (5000, r.p.m., 5 min). Pelleted cells and pulverized tissues were lysed in 100 μl 1% SDS lysis buffer and sonicated to 300–500 bp using a Bioruptor (Diagenode). ChIP was performed using the following antibodies: H3K4me3 (07-473, Millipore); H3K4me1 (ab8895, Abcam); H3K27ac (ab4729, Abcam). After recovery of ChIP and input DNA, whole-genome-amplification was performed using the WGA4 kit (Sigma-Aldrich) and BpmI-WGA primers. Amplified DNAs were purified using PCR purification columns (QIAGEN) and digested with BpmI (New England Biolabs) to remove WGA adapters. Thirty nanograms of amplified DNA was used for each sequencing library preparation (New England Biolabs). Eight libraries were multiplexed (New England Biolabs) and sequenced on two lanes of Hiseq2500 (Illumina) to an average depth of 20–30 million reads per library. Sequence mapping and ChIP-seq density analysis Sequence reads were mapped against human reference genome (hg19) using Burrows-Wheeler Aligner (BWA-MEM, version 0.7.0), after trimming the first and the last ten bases prior to alignment. Only high-quality mapped reads (MAPQ≥10) were retained for downstream analyses. The MAPQ value (≥10) was chosen as this has (i) been previously reported to be a good value to use for good/confident read mapping [71] ; (ii) MAPQ≥10 has also been indicated by the developers of the BWA-algorithm to be a suitable threshold to use for confident mappings using their software [72] ; and (iii) studies assessing various algorithms for read alignment have also shown that mapping quality scores do not correlate well with the likelihood of read mapping being true/accurate and have shown that the level of accuracy obtained for mapping accuracy plateaus between a 10–12 MAPQ threshold [73] . We also note that in our study we have focused on recurrent predicted enhancers and super-enhancers that are reliably detected in multiple samples, which increases the robustness of our analysis. Sequencing coverage was computed using MEDIPS with a 50 bp window size and read length extension to 200 bp. Peaks with significant ChIP enrichment (FDR<5%) relative to input libraries were detected using CCAT (version 3). Peak densities within a region were computed by counting the total number of mapped reads normalized by the library and region size, a metric equivalent to reads per million mapped reads per kilobases (RPKM). This normalization method adjusts for biases due to the higher probability of reads falling into longer regions and has been applied in previous studies [74] . We thus elected to apply RPKM-based normalization to make our study comparable to these other studies. To account for background signals, read densities of each ChIP library were corrected against the corresponding input library. Read densities across samples were corrected for potential batch effects (for example, date of ChIP assay) using COMBAT and to ensure equal sample variation. Of 17,360 recurrent predicted enhancers detected in two or more cell lines, 98% were present in at least one primary sample (normal or GC). Quality control assessment of nano-ChIPseq data We assessed qualities of the ChIP libraries (H3K27ac, H3K4me3 and H3K4me1) using two different methods. First, we estimated ChIP qualities, particularly H3K27ac and H3K4me3, by interrogating their enrichment levels at annotated promoters of protein-coding genes. Specifically, we computed median read densities of input and input-corrected ChIP signals at 1,000 promoters associated with highly expressed protein-coding genes. For each sample, we then compared read density ratios of H3K27ac over input as a surrogate of data quality, retaining only those samples where the H3K27ac/input ratio was greater than four-fold. Using these criteria, 48 out of 50 H3K27ac samples (GC lines and primary samples) exhibited greater than four-fold enrichment, indicating successful enrichment. A similar analysis was also performed for the H3K4me3 libraries (a promoter mark), and all 42 libraries satisfied this quality control criteria. Second, we used CHANCE (CHip-seq ANalytics and Confidence Estimation) [22] , a software for ChIP-seq quality control and protocol optimization that indicates whether a library shows successful or weak enrichment. We found that the large majority (85%) of samples in our study exhibited successful enrichment as assessed by CHANCE. The assessment status for each library, as assessed by both methods, are reported in Supplementary Data 1 . We experimentally generated a second biological replicate of H3K27ac Nano-ChIP-seq using KATO-III cells, and also compared our results against independent H3K27ac KATO-III data generated from regular ChIP-seq protocols [23] . The published sequencing reads were processed similarly to our NanoChIP-seq libraries, excluding sequence trimming. Peaks detected by CCAT at a FDR <5% were compared. Chromatin accessibility and binding enrichment Chromatin accessibility profiles of Epigenome Roadmap normal gastric tissues were obtained from the Gene Expression Omnibus (GSM1027325, GSM1027320) [28] . Read densities of chromatin accessibility profiles were computed for predicted enhancer regions and compared against 100,000 randomly selected regions in RPKM units. We also computed fractions of predicted enhancers overlapping open chromatin regions (.narrowPeak) and active regulatory elements (H3K27ac, .gappedPeak) from 25 Roadmap chromatin accessibility and H3K27ac profiles. For TF binding enrichment analysis, P300 and other TF binding coordinates curated by the ENCODE (wgEncodeRegTfbsClusteredV3.bed), were downloaded from the UCSC genome browser. Overlaps of at least 1 bp were identified using BEDTools intersect. Levels of evolutionary sequence conservation were assessed using PhastConst scores (Castelo R. phastCons100way.UCSC.hg19: UCSC phastCons conservation scores for hg19. R package version 3.2.0). The maximum score within 500 bp from the enhancer midpoint was used as the enhancer conservation score [75] . Conservation scores were also computed for 10,000 randomly selected regions, excluding pre-detected enhancer regions. Identification of predicted super-enhancers Predicted enhancers were defined as enriched H3K27ac regions at least 2.5 kb from annotated TSS and also showing enrichment of H3K4me1 and depletion of H3K4me3 (ref. 6 ). TSS annotations for this study were derived from GENCODE version 19. H3K4me3/H3K4me1 log ratios were computed using aggregated H3K4me3 and H3K4me1 signals from GC cell lines and primary samples. Distal predicted enhancers exhibiting high H3K27ac signals, but exhibiting high H3K4me3/H3K4me1 log ratios (>2.4, ref. 26 ) were classified as mistaken predictions and thus excluded from analyses. Predicted enhancers were then further subdivided into predicted super-enhancers or typical enhancers using the ROSE algorithm. Predicted super-enhancer regions with at least one base overlap across multiple GC lines were merged using BEDTools, and predicted enhancers localizing to regions distinct from the predicted super-enhancer regions were termed predicted typical enhancers. The presence of predicted typical or predicted super-enhancers in individual samples was determined by the level of H3K27ac enrichment above background ( P <0.01, empirical test), the latter being the H3K27ac signal (in RPKM) from 100,000 randomly selected regions. To assign predicted enhancers/super-enhancers to genes, we calculated distances from the predicted enhancer/super-enhancer centre to the nearest active TSS, defined as a promoter (500 bp flanking at TSS) with H3K27ac enrichment above randomly chosen regions [11] . Genes associated with recurrent predicted super-enhancers were tested for oncogene enrichment using a one-sided Fisher’s exact test. The top 500 oncogenes [76] were used. To identify recurrent predicted enhancer and predicted super-enhancers, the regions in each GC line were ranked according to signal strength. The ranks of each predicted enhancer/super-enhancer across the lines were multiplied to compute the rank product. To determine the statistical significance of the rank product, we compared the observed rank product against a null distribution—ranks in each line were reshuffled and the rank products computed. The reshuffling procedure was repeated for 10,000 iterations. Observed rank products less than the null distribution were considered statistically significant. Validation of predicted interactions Super-enhancer/gene assignments were validated using three orthogonal interaction data sets. These included: i Predetermined interactions detected by PreSTIGE [30] from 12 cell lines. PreSTIGE interaction data were downloaded from the PreSTIGE website (prestige.case.edu), involving cis -regulatory elements and target genes. ii cis -regulatory elements/gene assignment by GREAT [31] using the default parameters. iii Reference sets of enhancer-promoter interactions from RNAPII ChIA-PET studies in K562, HCT-116, NB4, MCF-7, HeLa-S3 and GM12878 cells. ChIA-PET interaction data were downloaded from encodeproject.org and GSE72816. All interactions identified in each biological replicate were considered for validation. These interactions involved two loci (anchors), one of which is within 2.5 kb of a TSS and the other anchor overlapping predicted super-enhancer regions found in our study. Besides (i)-(iii), additional validation was performed using Capture-C analysis on GC lines (see Fig. 4 of the Main Text). Functional enrichment analysis We used GOrilla [32] to identify biological processes (Gene Ontology annotations) enriched in recurrent predicted super-enhancer/gene promoter or predicted typical enhancer/gene promoter interactions. Default GOrilla parameters were used, and genes from GENCODE v19 were used as background. To ensure comparability, predicted typical enhancers with the highest H3K27ac across cell lines were selected to match the same number of recurrent predicted super-enhancers. To select the former, predicted typical enhancers were ranked in each line and were chosen based on the rank product score. The most significant terms (> 1.5-fold enrichment) associated with the recurrent predicted super-enhancers were then compared against enrichment levels associated with the top predicted typical enhancers. Besides GOrilla, we also studied functional enrichments associated with recurrent predicted super-enhancers and top predicted typical enhancers using GREAT using default parameters, as GREAT provides correction against genes flanked by larger intergenic regions [31] . Significant terms (also with >1.5-fold enrichment) were ordered based on Binomial P -values. Cell-line-derived super-enhancers in primary samples Regions showing H3K27ac enrichment or depletion of by two-fold or greater and with absolute differences of greater than 0.5 RPKM [4] were considered differentially present between GCs and matched normal samples. For PCA, we used signals from predicted super-enhancers showing somatic gain in two or more patients. PCA analysis was performed using R and plotted using the ‘pca3d’ package. We estimated the required sample size to achieve 80% power and 5% type I error ( http://powerandsamplesize.com/ ) based on the average signals of 100 predicted super-enhancers ( Supplementary Data 2 ) from tumour and normal samples. This result yielded a recommended sample size of 13 (average), which is met in our study (19N/T). Three classes of predicted super-enhancers were defined based on the primary samples: (i) somatic gain, (ii) somatic loss and (iii) unaltered. Genes associated with (i), (ii) and (iii) were mapped to gene groups previously reported in Hnisz, 2013 (ref. 11 ), where each group is a compilation of several gene ontology categories and used as a proxy for various cancerous hallmarks [11] . Statistical significance was computed using one-sided Fisher’s exact test in R. To assess lineage-specificities of the recurrently gained somatic predicted super-enhancers across different tissue types, we computed overlaps between the gastric predicted super-enhancers against other non-gastric tissues [11] . An enrichment ratio with each non-gastric tissue was computed based on the total observed overlap versus the total overlap by chance. Capture-C and data analysis Capture-C was performed as previously described [36] . Briefly, 1 × 10 7 cells were crosslinked by 2% formaldehyde, followed by lysis, homogenization, DpnII digestion, ligation and de-crosslinking. DNA was sonicated using a Covaris to 150–200 bp to produce DNA suitable for oligo capture. Three micrograms of sheared DNA was used for sequencing library preparation (New England Biolabs). Predicted super-enhancer sequences were double captured by sequential hybridization to customized biotinylated oligos (IDT, Supplementary Data 5 ) and enrichment with Dynabeads (LifeTech). Captured DNA was sequenced on an Illumina MiSEQ using the 150 bp paired-end configuration. Preprocessing of raw reads was performed to remove adaptor sequences (trim_galore, http://www.bioinformatics.babraham.ac.uk/projects/trim_galore/ ) and overlapping reads were merged using FLASH. In order to achieve short read mapping to the hg19 reference genome, the resulting preprocessed reads were then in-silico digested with DpnII and aligned using Bowtie (using p1, m2, best and strata settings). Aligned reads were processed using Capture-C analyser [36] to (i) remove PCR duplicates, and (ii) classify subfragments as ‘capture’ if they were contained within the capture fragment; ‘proximity exclusion’ if they were within 1 kb on either side of the capture fragment; or ‘reporter’ if they were outside of the ‘capture’ and ‘proximity exclusion’ regions. We additionally used the r3Cseq package [37] on the capture and reporter fragments to identify significant interactions of the viewpoint against a scaled background ( Q <0.05, FDR) and also to compare interaction profiles between different cell lines. 4C-seq and data analysis 4C templates were prepared using previously published protocols with slight modifications [77] . In brief, cultured cells were diluted into single-cell suspensions, and chromatin was cross-linked with 1% formaldehyde for 10 min at room temperature. Cells were lysed and cross-linked DNA was digested with the primary restriction enzyme HindIII-HF [R3104L, New England Biolabs (NEB)]. Next, HindIII-digested DNA was subjected to proximity ligation using T4 DNA ligase (EL0013, Thermo Scientific), followed by cross-link removal using Proteinase K (AM2546, Ambion), yielding 3C libraries. The 3C libraries were then subjected to a second restriction enzyme digestion using DpnII (R0543L, NEB), followed by a circularization reaction using T4 DNA ligase. For each viewpoint, 3.2 μg of the resulting 4C templates was used to perform a scale-up inverse, nested PCR ( Supplementary Table 5 ), of which 32 reactions (100 ng in each) were pooled and purified using the MinElute PCR Purification kit (Qiagen). Ten micrograms of the PCR products were then run on 4–20% TBE PAGE gels (5 μg per well). On the gel, smears from 200 to 600 bp were excised and unwanted PCR product bands were removed. DNA was then extracted from the cut-out gel pieces for next-generation sequencing on an Illumina Miseq (2 × 250 bp). Inverse primers were designed based on a viewpoint concept. The UCSC Genome Browser (assembly: Feb. 2009 (GRCh37/hg19)) was used to locate the region of interest. Upon addition of HindIII and DpnII tracks, two HindIII restriction sites flanking the region of interest were identified and the sequence between the nearest HindIII and DpnII restriction sites were selected as the viewpoint region. Based on this region, two pairs of primers (outer and nested) were designed using the Primer-BLAST program (National Center for Biotechnology Information (NCBI)) with the following adaptations to the default settings: optimal primer melting temperature of 58 °C, with a minimum of 55 °C and maximum of 60 °C; GC content between 39 and 60%. Appropriate adaptors (Nextera Index Kit—PCR primer, Nextera transposase sequence) and index sequences were then added to the nested primer pair. Outer and nested primers used in this study are presented in Supplementary Tables 4 and 5 respectively. Primer sequences at the 5′ ends of sequencing reads were trimmed using TagDust2, and mapped to the reference genome (hg19) using Bowtie2 (2.2.6). Unaligned reads were trimmed at the first 50 base pairs before realigning them to the reference genome. Only uniquely mapped reads with MAPQ≥30 were used in downstream analyses. Statistical significant interactions ( Q <0.05, FDR) were detected using r3Cseq using a non-overlapping window approach (window size=5 kb). Signal plots of 4C data were generated using Basic4CSeq. Detected interactions within DNA amplified regions were excluded. Interactions were then mapped to genes, using promoters (+/− 2.5 kb from annotated TSSs from GENCODE v19) overlapping with the interactions. CRISPR/Cas9 enhancer deletions CRISPR sgRNA target search was performed using online software created by the Feng Zhang laboratory ( http://tools.genome-engineering.org ). sgRNA pairs were designed to target sequences flanking enhancers identified for deletion. Briefly, sequences corresponding to 100 bp upstream/20 bp downstream of the 5′ end of the enhancer, and sequences corresponding to 20 bp upstream/100 bp downstream of the 3′ end of the enhancer, were used for the search. Top hits with the lowest level of coding region off-target predictions were chosen. sgRNAs were cloned into the pSpCas9(BB)-2A-GFP or -Puro vectors (Addgene). Briefly, pairs of oligonucleotides were designed and procured from Integrated DNA Technologies, Inc. for each CRISPR target. Oligonucleotide pairs were then annealed to form DNA duplexes containing overhangs on both sides for ease of cloning. Guide RNAs used to target 5′ ends of individual enhancers were cloned into Bbs I-digested pSpCas9(BB)-2A-GFP vectors, while sgRNAs targeting 3′ ends of each enhancer were cloned into Bbs I-digested pSpCas9(BB)-2A-Puro vectors. The inserts and vectors were ligated using T4 DNA Ligase (New England Biolabs). DH5α cells were transformed with the ligation product and plated on LB agar supplemented with ampicillin. Colonies were picked and cultured, and plasmids extracted using the Wizard Plus SV Minipreps DNA Purification System (Promega). Sequences of plasmids were confirmed by performing Sanger sequencing. Oligonucleotides used for these experiments are listed in Supplementary Table 6 . SNU16 and OCUM-1 cells were grown to 80–90% confluence in Roswell Park Memorial Institute (RPMI) supplemented with 10% fetal bovine serum (FBS), 1xP/S and 0.5XNEAA. Cells were harvested and spun down, treated with Typsin for 5 min at 37 degrees, and re-suspended by pipetting to achieve single cell suspensions. Cell numbers were counted, and cells were washed once with 1 × PBS before resuspension in Resuspension buffer (R) at 1 × 10 7 cells/ml. For every 1 × 10 7 cells in 1 ml of Resuspension buffer, 25 μg of pCas9-GFP-sgRNA and 25 μg of pCas9-Puro-sgRNA plasmid were mixed with SNU16 or OCUM-1 cells. Hundred microlitres of each cell suspension was electroporated using a 100 μl Neon pipette in a Neon tube containing 3 ml of Electrolytic Buffer (E2). Electroporation conditions were: Pulse, V 1050, MS 30, Number 2. After electroporation, cells were plated onto 8 ml of RPMI supplemented with 10% FBS, 1xP/S and 0.5XNEAA. At 24 h after initial transfection, the cells were treated with 10 μg of Puromycin for 48 h, and the remaining GFP-positive cells were sorted using FACS. The remaining surviving cells (both GFP-positive and Puromycin-resistant) were then subsequently analysed using qPCR to estimate knockout efficiencies. We performed quantitative PCR (qPCR) to determine the efficiency of deletion of individual enhancers in CRISPR/Cas9-targeted cells. Genomic DNA of targeted and untargeted cells (pooled) was extracted using the AllPrep DNA Micro Kit (QIAGEN) and subjected to qPCR in technical triplicates using KAPA SYBR FAST qPCR Master Mix (Kapa Biosystems) on a CFX96 Touch Real-Time PCR Detection System (Bio-Rad Laboratories, Inc.). Primers used in these reactions are listed in Supplementary Table 6 (primers with ‘Int’ in their names were used for this purpose). Relative amount of the specific targeted region present in the genomic DNA samples was calculated using the comparative C T (ΔΔC T ) method, normalized to the GAPDH gene and relative to untargeted cells. Genomic DNA was extracted from the sorted cells using a previously described protocol [78] . Briefly, cells were triturated in 0.5 × Direct-Lyse buffer (10 mM Tris pH 8.0, 2.5 mM EDTA, 0.2 M NaCl, 0.15% SDS, 0.3% Tween-20) and subjected to the following heating and cooling program: 65 °C for 30 s, 8 °C for 30 s, 65 °C for 1.5 min, 97 °C for 3 min, 8 °C for 1 min, 65 °C for 3 min, 97 °C for 1 min, 65 °C for 1 min and 80 °C for 10 min. Subsequently, the lysates were diluted approximately 4 × in water and 3 μl of the diluted lysates were used to perform 20-μl PCR reactions using Taq DNA Polymerase (Life Technologies). Primers used are in Supplementary Table 6 (primer pairs of ‘5′ F’ and ‘3′ R’ for each enhancer). RT-qPCR to measure gene expression levels . Cells were FACS sorted for GFP-positive cells and total RNA was extracted from cells using AllPrep DNA/RNA Micro Kit (QIAGEN). Reverse transcription was performed on pooled cells using iScript Select cDNA Synthesis Kit (Bio-Rad) with random primers. qPCR was conducted using TaqMan Gene Expression Master Mix and TaqMan probes (Applied Biosystems) on a CFX384 Touch Real-Time PCR Detection System (Bio-Rad). All qPCR experiments were run in triplicate, and mean values were used to determine mRNA levels. Relative quantification was performed using the comparative C T method with GAPDH as the reference gene and with the formula 2-ΔΔC T . Copy number alterations and DNA methylation Genomic DNAs from gastric tumours and matched normal gastric tissues were hybridized on Affymetrix SNP6.0 arrays (Affymetrix, Santa Clara, CA). Data in CEL format was processed in the following order: (1) Normalization: Raw.CEL files were processed using Affymetrix Genotyping Console 4.2. Reference models were created from SNP6.0 profiles of normal gastric tissues according to the hybridization batch. Copy number changes in cell lines and primary tumour samples were determined by using the reference model from primary normal samples. (2) Segmentation: Copy number segmentation data were produced using the circular binary segmentation (CBS) algorithm implemented in the DNAcopy R package. The P -value cutoff for detecting a change-point was 0.01, with a permutation number of 10,000. Copy number gain and loss regions were defined for showing average log ratios of >0.6 and<−1.0, respectively. Illumina HumanMethylation450 (HM450) Infinium DNA methylation arrays were also used to assay DNA methylation levels. Methylation β-values were calculated and background corrected using the methylumi R BioConductor package. Normalization was performed using the BMIQ method (watermelon package in R). RNAseq and analysis Total RNA was extracted using the Qiagen RNeasy Mini kit. RNA-seq libraries were constructed according to manufacturer’s instructions using Illumina Stranded Total RNA Sample Prep Kit v2 (Illumina, San Diego, CA) Ribo-Zero Gold option (Epicentre, Madison, WI) and 1 μg total RNA. Completed libraries were validated with an Agilent Bioanalyzer (Agilent Technologies, Palo Alto, CA) and applied to an Illumina flow cell via the Illumina Cluster Station. Sequencing was performed using the paired-end 101 bp read option. RNA-seq reads were aligned to the human genome (hg19) using TopHat2-2.0.12 (default parameter and --library-type fr-firststrand). The per base sequence quality and per sequence quality scores of the mapped reads was assessed using FastQC version 0.10.1 ( http://www.bioinformatics.babraham.ac.uk/projects/fastqc/ ). Transcript abundances at the gene level were estimated by cufflinks. Gene expression from primary samples showing variation greater than zero was corrected for potential batch effects using ComBat. Gene expression values were measured in FPKM units. Differential expression between groups was identified as genes showing altered expression by at least two-fold and absolute differences of 0.5 FPKM. Survival analysis GC samples from seven independent studies were clustered using a K-medoids approach. Only genes with expression values in all seven studies were used in analyses. Kaplan–Meier survival analysis was employed with overall survival as the outcome metric. Log-rank tests were used to assess the significance of Kaplan–Meier curves. Multivariate analysis involving additional variables, such as age, tumour stage, Lauren’s histological subtypes and locality (Asian versus Non-Asian), was performed using Cox regression. Disease-associated SNP analysis Trait-associated SNPs were downloaded from the UCSC browser of GWAS (27 August 2015). For this study, we focused on SNPs occurring in noncoding regions and excluded SNPs within coding regions. We computed overlaps between SNPs from each trait/disease and somatic predicted super-enhancers using BEDtools ‘intersect’ (nGWAS), and compared nGWAS against the total number of disease-associated SNPs outside the predicted super-enhancers (nGWAS’). As an additional control, we created an ‘SNP background’ model using a set of all SNPs from two commonly used SNP arrays (Illumina HumanHap550 and Affymetrix SNP6). The number of SNPs from the SNP background overlapping the predicted super-enhancers was calculated (nBackground) and compared against the total number of background SNPs outside the predicted super-enhancers (nBackground′). The ratio of normal SNPs in predicted super-enhancers was computed as nBackground/nBackground′. Expecting that the increased number of disease-associated SNPs in predicted super-enhancers is associated with a high prevalence of SNPs in these regions, our null hypothesis is therefore that there is no difference between the ratio of disease-associated SNPs and the ratio of normal SNPs (enrichment ratio). Chi-square tests were conducted, with enrichment P -values of<0.01 considered statistically significant. To understand the relationship between risk-associated SNPs and histone modification, we identified validated SNPs in gastrointestinal diseases (for example, ulcerative colitis and colorectal cancer) found to be associated with disease in at least two independent studies. Samples were classified into two groups based on the presence of the disease-associated SNPs, using GATK Unified Genotyper. Differences of H3K27ac signals between tumour and matched normal in samples with or without disease-associated SNPs were compared. TF binding motif analysis We interrogated enrichments of TFs in somatic gain predicted super-enhancers and unaltered predicted super-enhancers using the ReMap database [48] . Transcription factor binding sites with at least 60% of overlap with predicted super-enhancers were counted, and the ranks of the top 10 most enriched TFs compared. Binding densities of TFs were computed as the total binding sites detected in the regions divided by the total size of the regions in unit of million base pairs (Mbp). For CDX2, we examined CDX2 binding sites in recurrently gained somatic predicted super-enhancers to predict nearby binding of other TFs, using HOMER with default parameters [49] . The top 20 TF identified from the HOMER outputs were used for expression correlation analysis. Additionally, we also identified CDX2 co-binding motifs using PScanChIP [50] with JASPAR 2016. Expression correlations (Spearman’s correlation) between CDX2 and potential co-binding partners were evaluated. siRNA transfection ON-TARGETplus Human siRNA SMARTpools ( HNF4α and CDX2) , individual ON-TARGETplus Human individual siRNAs ( HNF4α) and ON-TARGETplus Non-targeting siRNA controls (Dharmacon/Thermo Fisher Scientific) were used to transfect cells (2 × 10 5 ) at 50 nM in 6-well plate, using Dharmafect 1 transfect reagent, according to the manufacturer instructions. Knockdown efficiency after 72 h RNAi treatment was examined using quantitative RT-PCR and/or Western Blot analysis ( Supplementary Fig. 17 ). Western blotting Cells (2 × 10 5 ) were harvested in RIPA buffer (Sigma) and lysed for 10 min on ice. Concentration of supernatants was measured using Pierce BCA protein assay (Thermo Scientific). CDX2 (1:500; MU392A-UC, Biogenex), HNF4α (1:1,000; sc-8987, Santa Cruz Biotechnology) and GAPDH (1:3,000; 60,004-1-Ig, Proteintech Group) antibodies were used to probe the lysate. Quantitative RT-PCR Total RNA was isolated using RNeasy Mini Kit (Qiagen), and DNA was removed using RNase-Free DNase Set (Qiagen). Two micrograms RNA was reverse transcribed using Superscript III First Strand Synthesis System (Invitrogen), and complementary DNA was amplified using SYBRGreen PCR Master Mix (Applied Biosystems). Fold changes were normalized to GAPDH . Primer sequences are as follows: HNF4α: F1-5′ GTGCGGAAGAACCACATGTACTC 3′, R1-5′ CGGAAGCATTTCTTGAGCCTG 3′, F2-5′ CTGCAGGCTCAAGAAATGCTT 3′, R2-5′ TCATTCTGGACGGCTTCCTT 3′, F3-5′ TGTCCCGACAGATCACCTC 3′, R3-5′ CACTCAACGAGAACCAGCAG 3′; CDX2: F1-5′ GCAGCCAAGTGAAAACCAGG 3′, R1-5′ CCTCCGGATGGTGATGTAGC 3′, F2-5′ AGTCGCTACATCACCATCCG 3′, R2-5′ TTCCTCTCCTTTGCTCTGCG 3′; GAPDH: F-5′ CCAGGGCTGCTTTTAACTC 3′, R-5′ GCTCCCCCCTGCAAATGA 3′. CDX2 and HNF4α ChIP-seq and analysis Cells were cross-linked with 1% formaldehyde for 10 min at room temperature, and stopped by adding glycine to a final concentration of 0.2 M. Chromatin was extracted and sonicated to 500 bp. CDX2 (MU392A-UC, Biogenex) and HNF4α (sc-8987, Santa Cruz Biotechnology) antibodies were used for chromatin immunoprecipitation (ChIP). ChIPed DNA (10 ng) was used for ChIP with DNA sequencing (ChIP-seq) library construction following manufacturer protocols (New England Biolabs). Input DNA from cells prior to immunoprecipitation was used to normalize ChIP-seq peak calling. Prior to sequencing, qPCR was used to verify that positive and negative control ChIP regions amplified in the linear range. Size distributions of the library samples were checked using a Bio-analyzer (Agilent Technologies). In an initial analysis comparing recurrently gained predicted super-enhancers specific to intestinal and diffuse-type GCs (10 intestinal, 6 diffuse), we did not observe any significant differences in CDX2 binding between the two subtypes. A deeper analysis revealed, however, high within-subtype variability in CDX2 expression between individual tumours of the same subtype, consistent with previous reports that CDX2 expression is not absolutely associated with intestinal subtype GC [79] . We thus performed a complementary analysis where the GCs were ordered by their individual CDX2 expression levels and examined. CDX2 binding density were then computed at recurrent somatic gain predicted super-enhancers identified in GC samples showing high ( n =8) and low ( n =8) CDX2 expression. In differential binding signal analysis, we computed binding signals for CDX2 and HNF4α for 200 bins spanning those predicted super-enhancers showing somatic gain or no alteration in primary samples and also detected in OCUM-1 or SNU16 cell lines. Signals were measured in RPKM units. To estimate the effect of TF knockdown on H3K27ac strength, we defined an internal control comprising observed variation of H3K27ac signals between independent wild-type (WT) samples. We then measured differences between WT samples against TF-silenced (siCDX2, siHNF4α, or double TF) samples, which were then compared against this background variation. Subregions with differences>99% of background variation were termed as H3K27ac depletion; while differences<1% of the background variation were termed as H3K27ac gain. Statistical enrichments of H3K27ac-depleted subregions corresponding to predicted super-enhancers were conducted using one-sided Fisher’s exact test. To study relationships between the differential regions and their distances to nearby CDX2/HNF4α binding sites, the regions were also segregated into three categories (near, moderate, distal) based on their distance distribution. Mid-point locations between the CDX2 and HNF4α summits were used to analyse distances between H3K27ac-depleted subregions and CDX2-HNF4α cobinding sites. To study associations between gene expression and somatic gain predicted super-enhancers in TF-silenced cells, we selected genes linked to predicted super-enhancers exhibiting significant positive expression correlations with H3K27ac predicted super-enhancer signals in primary samples ( r >0.4; P <0.05, two-sided t -test) and also observed in the GC cell lines. To assess the significance of TF knockdown on predicted super-enhancer target gene expression, we used a permutation approach. Specifically, focusing on predicted super-enhancers exhibiting H3K27ac depletion after TF silencing, we permuted the actual super-enhancer to gene assignments 10,000 times. An empirical P -value was then derived by counting the number of times the number of downregulated genes in the permuted gene/super-enhancer set exceeded the experimentally observed number of downregulated genes in the actual gene/super-enhancer set. Data availability Histone NanoChIP-seq (GSE76153 and GSE75898), SNP array (GSE85466), RNA-seq (GSE85465) and DNA methylation data (GSE85464) generated during this study have been deposited in Gene Expression Omnibus. Previously deposited histone ChIP-seq (GSE51776 and GSE75595) and SNP array (GSE31168 and GSE36138) data that are used in this study are available in Gene Expression Omnibus. Chromatin accessibility profiles of normal gastric tissues from Epigenome Roadmap were obtained from the Gene Expression Omnibus (GSM1027325, GSM1027320). RNAPII ChIA-PET data analysed in this study was obtained from encodeproject.org and Gene Expression Omnibus (GSE72816). The authors declare that all other data are available within the Article or associated Supplementary information files , or available from the author on request. How to cite this article: Ooi W. F. et al . Epigenomic profiling of primary gastric adenocarcinoma reveals super-enhancer heterogeneity. Nat. Commun. 7:12983 doi: 10.1038/ncomms12983 (2016).